Atomically precise edge chlorination of nanographenes and its application in graphene nanoribbons Chemical functionalization is one of the most powerful and widely used strategies to control the properties of nanomaterials, particularly in the field of graphene. However, the ill-defined structure of the present functionalized graphene inhibits atomically precise structural characterization and structure-correlated property modulation. Here we present a general edge chlorination protocol for atomically precise functionalization of nanographenes at different scales from 1.2 to 3.4 nm and its application in graphene nanoribbons. The well-defined edge chlorination is unambiguously confirmed by X-ray single-crystal analysis, which also discloses the characteristic non-planar molecular shape and detailed bond lengths of chlorinated nanographenes. Chlorinated nanographenes and graphene nanoribbons manifest enhanced solution processability associated with decreases in the optical band gap and frontier molecular orbital energy levels, exemplifying the structure-correlated property modulation by precise edge chlorination. Graphene, a monolayer of carbon atoms arranged in a honeycomb network, has attracted immense interest [1] , [2] due to its extraordinary physical properties, which are governed by the size of the sheet and the nature of its periphery [3] , [4] , [5] , [6] . Chemical functionalization can further modify the chemical and physical properties of graphene and typically follows two approaches [6] , [7] , [8] : functionalization on the basal plane of graphene via covalent addition to C=C bonds or at the edge via the replacement of peripheral hydrogen atoms with functional groups. Precise edge functionalization is a long-sought and appealing strategy towards controllable manipulation of the physical properties of graphene [9] , [10] , [11] , [12] . However, the established chemical functionalization protocols for graphene, such as Friedel–Crafts reaction, diazonium salt addition and so on fail to reach the atomic accuracy required for reliable structure–property correlations [13] , [14] , [15] , [16] . Here we report a general and simple edge chlorination protocol for graphenes by electrophilic substitution. Using this strategy, we successfully achieve atomically precise chlorination of a series of nanographenes with carbon numbers ranging from 42 to 222, corresponding to a molecular size of 1.2–3.4 nm, in high yields. By taking advantage of the pronounced solution processability, we are able to determine the structures of five chlorinated nanographenes by X-ray single-crystal diffraction. In comparison with pristine nanographenes, these chlorinated molecules show characteristic non-planar molecular geometry, which strongly influences their crystal packing. Extending to organic synthetic graphene nanoribbons (GNRs) with a width of 1.2 nm and approximate length of 390 nm, the efficient edge chlorination is also achieved. Both edge-chlorinated nanographenes and GNRs exhibit enhanced solubility, defined and tunable band gaps, as well as decreased frontier molecular orbital energy levels. Edge chlorination of well-defined nanographenes We chose a series of unique well-defined nanographenes (C 42 H 18 , C 48 H 18 , C 60 H 22 , C 60 H 24 , C 96 H 30 , C 132 H 34 and C 222 H 42 ; Supplementary Fig. S1 ) for atomically precise edge chlorination. These graphene molecules were obtained in our laboratories by cyclodehydrogenation of dendritic polyphenylene precursors [17] . In general, chlorination was accomplished in CCl 4 at 80 °C with excess iodine monochloride and catalysed by AlCl 3 . After quenching the reaction with ethanol, the precipitate was filtered and washed, providing chlorinated nanographenes (C 42 Cl 18 ( 1 ), C 48 Cl 18 ( 2 ), C 60 Cl 22 ( 3 ), C 60 Cl 24 ( 4 ), C 96 Cl 27 H 3 ( 5 ), C 132 Cl 30 H 2 ( 6 ) and C 222 Cl 42 ( 7 ) ( Fig. 1a )) in a yield of 83–97%. The elemental composition of chlorinated products 1 – 7 was confirmed by matrix-assisted laser desorption/ionization–time of fight mass spectrometry. As depicted in Fig. 1b , there was only one dominant peak in the respective mass spectra of 1 – 7 , revealing their defined molecular composition; the isotopic distribution pattern of the mass peak was in good agreement with the calculated patterns ( Supplementary Fig. S2 ), confirming the molecular formulae of 1 – 7 . The obtained compounds 1 – 7 were also analysed by thin-layer chromatography, high-performance liquid chromatography and infrared spectra ( Supplementary Figs S3–S5 ). A longer reaction time or higher reaction temperature did not lead to further chlorination or destruction of the products. Thus, the chlorination appears to occur selectively at the nanographene edge by electrophilic substitution, whereas chlorine substitution did not affect the sp 2 framework of nanographene under the reaction conditions. In contrast, previously reported chlorination of graphenes occurs by the addition of C=C bond on graphene plane [18] , [19] , [20] . 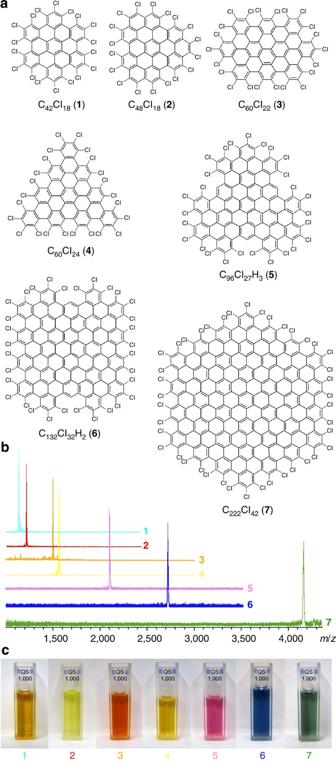Figure 1: Chlorinated nanographenes (1–7). (a) Structural formulae; (b) mass spectra; (c) photos of the toluene solution of1–7. Figure 1: Chlorinated nanographenes (1–7). ( a ) Structural formulae; ( b ) mass spectra; ( c ) photos of the toluene solution of 1 – 7 . Full size image Interestingly, in contrast to the complete edge chlorination in the case of 1 – 4 and 7 , three and two hydrogen atoms remained in 5 and 6 , respectively, after the chlorination reaction ( Fig. 1a ). The number of unreacted hydrogens was exactly the same as that in the gulf regions [21] ( Supplementary Fig. S6 ) in 5 and 6 . Remarkably, we were able to record the 1 H NMR spectrum of 5 in 1,1,2,2-tetrachloroethane- d 2 , which is the largest nanographene measured by 1 H NMR to date ( Supplementary Fig. S7 ). We assume that the hydrogen atoms in the gulf region cannot be replaced because of the steric hindrance induced by the neighbouring substituted chlorines. In comparison with the insoluble nature of parent nanographenes with hydrogen termination [22] , [23] , chlorinated molecules 1 – 7 can be readily dissolved to form homogeneous solutions in common organic solvents such as toluene, chloroform and carbon disulphide ( Fig. 1c ; typical concentrations of saturated carbon disulphide solutions of 1 – 7 range from 4.0 to 0.2 mg ml −1 ). Therefore, taking advantage of the increased solubility and the well-defined chemical structures, we grew single crystals of 1 – 5 by solvent evaporation. The structures of 1 – 5 were unequivocally characterized by X-ray diffraction, as depicted in Fig. 2 . Compound 5 with a molecular size of 2.0 nm is the largest nanographene so far characterized crystallographically. 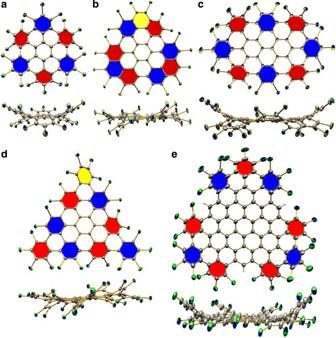Figure 2: Crystal structures of chlorinated nanographenes (1–5). (a) C42Cl18(1); (b) C48Cl18(2); (c) C60Cl22(3); (d) C60Cl24(4); and (e) C96Cl27H3(5). Front- and side-view representations of the structures of1–5are shown. The ORTEP drawings show thermal ellipsoids at a 50% probability level. The carbon and chlorine atoms are represented as grey and green balls, respectively. The peripheral hexagons flip up and down with respect to the inner rings, which are highlighted in blue and red, respectively. The hexagons in2and4, which adopt the twisted configuration, are highlighted in yellow. Figure 2: Crystal structures of chlorinated nanographenes (1–5). ( a ) C 42 Cl 18 ( 1 ); ( b ) C 48 Cl 18 ( 2 ); ( c ) C 60 Cl 22 ( 3 ); ( d ) C 60 Cl 24 ( 4 ); and ( e ) C 96 Cl 27 H 3 ( 5 ). Front- and side-view representations of the structures of 1 – 5 are shown. The ORTEP drawings show thermal ellipsoids at a 50% probability level. The carbon and chlorine atoms are represented as grey and green balls, respectively. The peripheral hexagons flip up and down with respect to the inner rings, which are highlighted in blue and red, respectively. The hexagons in 2 and 4 , which adopt the twisted configuration, are highlighted in yellow. Full size image Structure analysis of 1–5 The crystal data on 1 – 5 ( Supplementary Data 1 and Supplementary Table S1 ) provide structural information that is relevant for understanding the bond length and structure evolution of two-dimensional infinite graphene [24] . Although the mean bond length of 1 – 5 ( Supplementary Table S2 ) is comparable to the fully equalized C–C bond value in infinite graphene (1.415 Å) [25] , two classes of C–C bonds can be distinguished for 1 and 3 – 5 . One C–C bond located in the benzenoid rings has a shorter mean length, whereas the longer bond connecting the benzenoid rings has more of a single-bond character ( Supplementary Table S2 ). This is consistent with the fully benzenoid description in terms of Clar’s sextet model [26] . With the increase of the π -system, however, there is a clear tendency towards equalization of the bond lengths in the interior of 5 (1.411–1.429 Å). Compound 2 with a partial zigzag edge is unique in that the bond lengths ( Supplementary Table S2 ) are more equalized and no sextet benzenoid rings can be assigned based on the distinction of bond lengths. This clearly exemplifies the influence of the periphery structure on the whole molecule. The olefinic bonds at edges of 1 – 5 are obviously shorter than those in their interior ( Supplementary Table S2 ) [24] , [27] , indicating a large polarization of the charge distribution at the periphery [28] . Compared with the hydrogen termination of parent nanographenes, the chlorine atoms of 1 – 5 induce severe steric hindrance and force the outer benzene rings of the carbon framework to flip up and down in an alternating manner ( Fig. 2 ). The curvature of the non-planar discs 1 – 5 can be quantified by the dihedral angles between the inner rings and the outside distorted ring ( β -angle), which are as large as 48°. This value is much larger than that (23.6°) of the bowl-shaped fullerene segment corannulene [29] . The theoretically optimized structures of 6 and 7 also show a non-planar molecular geometry ( Supplementary Fig. S8 ). Packing structure of 1–5 The non-planarity feature strongly influences the packing of chlorinated nanographenes. As revealed by crystallography, the major intermolecular interactions within the crystals of 1 – 4 comprise Cl– π and Cl–Cl short contacts without close π–π interactions ( Supplementary Figs S9–S12 and Fig. 3 ). As shown in Fig. 3a–d , the distance between the planes of adjacent molecules in crystal of 1 – 4 ranges from 3.95 to 6.00 Å, obviously larger than that of typical π–π stacking (3.30 Å). This is in contrast to the typical condensed polycyclic aromatic hydrocarbons that stack largely by π–π interactions [22] , [30] . Interestingly, as the molecular size increased, compound 5 forms dimmers with interlayer distance of 3.30 Å ( Fig. 3e ), showing obvious π–π interactions within the dimer. However, apart from the π–π interactions present in dimers, only Cl– π and Cl–Cl short contacts exist among these dimers ( Supplementary Fig. S13 ). The distorted edge structure of chlorinated nanographenes thus obstructs the π–π stacking, thereby enhancing the solubility of these molecules in common organic solvents. It is very likely to be that a similar conformational effect steers the solution processability of the edge-functionalized graphene materials [14] , [16] . 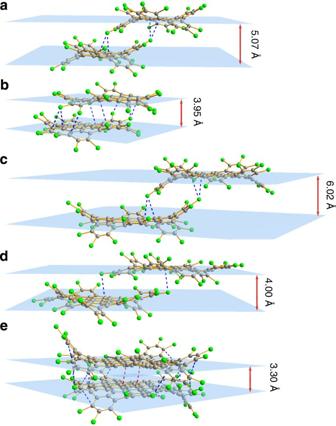Figure 3: Crystal packing of 1–5. (a) C42Cl18(1); (b) C48Cl18(2); (c) C60Cl22(3); (d) C60Cl24(4); and (e) C96Cl27H3(5). The Cl–πshort contacts are represented as blue dashed line. Theπ–πshort contacts in dimmer of5are represented as red dashed line. Figure 3: Crystal packing of 1–5. ( a ) C 42 Cl 18 ( 1 ); ( b ) C 48 Cl 18 ( 2 ); ( c ) C 60 Cl 22 ( 3 ); ( d ) C 60 Cl 24 ( 4 ); and ( e ) C 96 Cl 27 H 3 ( 5 ). The Cl– π short contacts are represented as blue dashed line. The π – π short contacts in dimmer of 5 are represented as red dashed line. Full size image Optical properties of chlorinated nanographenes The ultraviolet–visible–near-infrared optical absorption bands of 1 – 7 ( Fig. 4a ) are sharper and exhibit more abundant fine structures than those of alkyl-substituted counterparts [31] , suggesting less aggregation in solution. Time-dependent density functional theory (DFT) calculations indicate strong configurational mixing associated with near degeneracy of the frontier molecular orbitals (see Supplementary Methods for computation details and Supplementary Figs S14 and S15 ). More interestingly, the absorption bands of 1 – 7 show a bathochromic shift of 40–50 nm with respect to the hydrogen-terminated compounds [31] ( Supplementary Table S3 ), which are supported by the time-dependent DFT calculations. Thus, edge chlorination appears to be a powerful protocol for decreasing the optical band gap of nanographenes. In fact, a decrease in the optical gap is a consequence of the asymmetric stabilization of the frontier molecular orbitals when substituting hydrogens with electron-withdrawing chlorines (the effect is smaller for the highest occupied molecular orbital, where it is partly compensated by a mesomeric electron-donating effect). 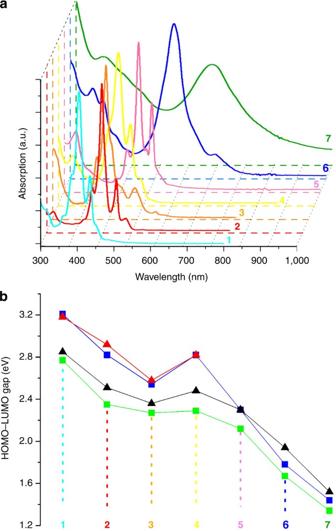Figure 4: Optical properties of chlorinated nanographenes. (a) Ultraviolet–visible–near-infrared spectra of1–7were acquired in toluene. The respective spectra are indicated by the corresponding Arabic numeral of the chlorinated nanographenes. (b) The calculated and experimental highest occupied molecular orbital–lowest unoccupied molecular orbital (HOMO–LUMO) gaps of1–7are represented by green squares and black triangles, and those of their hydrogen-terminated counterparts are represented by blue squares and red triangles, respectively. Figure 4: Optical properties of chlorinated nanographenes. ( a ) Ultraviolet–visible–near-infrared spectra of 1 – 7 were acquired in toluene. The respective spectra are indicated by the corresponding Arabic numeral of the chlorinated nanographenes. ( b ) The calculated and experimental highest occupied molecular orbital–lowest unoccupied molecular orbital (HOMO–LUMO) gaps of 1 – 7 are represented by green squares and black triangles, and those of their hydrogen-terminated counterparts are represented by blue squares and red triangles, respectively. Full size image Electronic properties of chlorinated nanographenes The electron-withdrawing effect of chlorines lowers the energetic position of the frontier molecular orbitals for all chlorinated nanographenes ( 1 – 7 ) by around 1.0 eV, in comparison with the respective hydrogen-terminated analogues ( Supplementary Fig. S16 and Supplementary Table S4 ). The calculated energy position of the lowest unoccupied molecular orbital in 1 – 7 spans from −3.37 to −4.01 eV, which is in the range of energy levels suited for electron injection in n -channel semiconductors [32] . This result indicates the potential use of chlorinated nanographenes as electronic acceptors in devices. Indeed, we found that the vacuum-deposited film of compound 4 (40 nm in thickness), despite the amorphous morphology on the surface, shows an obvious n -type transport behaviour, with a mobility of 1.0 × 10 −4 cm 2 V −1 s −1 and on/off ratio of 10 3 ( Supplementary Fig. S17 ). In contrast, the typical alkyl chain substituted nanographenes display p -type transport features [17] . Edge chlorination of GNRs Encouraged by the successful atomically precise edge chlorination for model nanographene systems <4.0 nm in size, we subjected organic synthetic GNRs ( Supplementary Fig. S18 ) to chlorination under similar reaction conditions. Such GNRs have a well-defined chemical structure ( Fig. 5a ) and a remarkably large aspect ratio (molecular weight around 260,000 Da, width of 1.2 nm and approximate average length of 390 nm). Tert -butyl groups were intentionally introduced at the edge periphery of GNRs during organic synthesis to impart reasonable solubility in common organic solvents. The tert -butyl groups can be readily replaced by chlorine atoms under the reaction conditions, based on a model reaction of hexa- tert -butyl-hexa- peri -hexabenzocoronene ( Supplementary Fig. S19 ). Thereby, the edge-chlorinated GNRs were obtained. By analogy, and supported by X-ray photoelectron spectroscopy (XPS) analysis and infrared spectroscopy, we proposed a structure of chlorinated GNRs as shown in Fig. 5a . 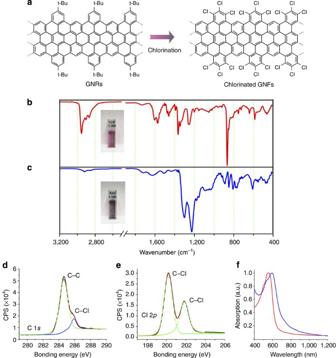Figure 5: Chlorination of bottom-up synthetic GNRs. (a) Scheme of chlorination of bottom-up synthetic GNRs. (b) Infrared spectrum of GNRs shows the vibrations of thetert-butyl group at 2,953, 1,364 and 866 cm−1. (c) Infrared spectrum of chlorinated GNRs shows the vibration peaks of C=C in chlorinated aromatic carbon at 1,299 and 1,225 cm−1and vibration peaks of C–Cl bonds at 810, 770 and 608 cm−1. (d) C 1sXPS of chlorinated GNRs. The XPS signal of C 1sat 284.6 and 285.9 eV. (e) Cl 2pXPS of chlorinated GNRs. The Cl 2ppeaks at 200.2 eV (2p3/2) and 201.8 eV (2p1/2). (f) Ultraviolet–visible–near-infrared spectra of GNRs (blue) and chlorinated GNRs (red) in 1,2,4-trichlorobenzene (TCB). Insert images are photos of GNRs and chlorinated GNRs solution in TCB, respectively. Figure 5: Chlorination of bottom-up synthetic GNRs. ( a ) Scheme of chlorination of bottom-up synthetic GNRs. ( b ) Infrared spectrum of GNRs shows the vibrations of the tert -butyl group at 2,953, 1,364 and 866 cm −1 . ( c ) Infrared spectrum of chlorinated GNRs shows the vibration peaks of C=C in chlorinated aromatic carbon at 1,299 and 1,225 cm −1 and vibration peaks of C–Cl bonds at 810, 770 and 608 cm −1 . ( d ) C 1 s XPS of chlorinated GNRs. The XPS signal of C 1 s at 284.6 and 285.9 eV. ( e ) Cl 2 p XPS of chlorinated GNRs. The Cl 2 p peaks at 200.2 eV (2 p 3/2) and 201.8 eV (2 p 1/2). ( f ) Ultraviolet–visible–near-infrared spectra of GNRs (blue) and chlorinated GNRs (red) in 1,2,4-trichlorobenzene (TCB). Insert images are photos of GNRs and chlorinated GNRs solution in TCB, respectively. Full size image After chlorination of GNRs, the vibrations of the tert -butyl group vanished and those of the C–H bond became much weaker ( Fig. 5b ). In addition, obvious vibration peaks of the C=C and C–Cl bonds in chlorinated aromatic carbon appeared ( Fig. 5c ). These spectral changes clearly demonstrated the successful replacement of the tert -butyl groups and hydrogen atoms of GNRs by chlorines. XPS analysis further confirmed the structure of chlorinated GNRs. High-resolution XPS scans for C 1 s and Cl 2 p peaks of chlorinated GNRs are shown in Fig. 5d,e , respectively. The bonding energy of Cl 2 p and C 1 s of chlorinated GNRs was the same as that of chlorinated nanographenes ( Supplementary Fig. S20 ), confirming the covalent bonding of the chlorine atoms to the carbon skeleton. On the basis of the peak area in Cl 2 p and C 1 s , the atomic ratio of carbon to chlorine was calculated to be about 4.5/1, which is close to the stoichiometric C/Cl ratio (5.0/1) expected for (C 30 Cl 6 H 2 ) n . Properties of chlorinated GNRs Similar with chlorinated nanographenes, edge chlorination can promote the solubility and, therefore, the processability of GNRs without the use of surfactant or long alkyl-chain decoration. Chlorinated GNRs can be dissolved in high polar solvents, such as N -methylpyrrolidone or highly polarizable solvent, such as 1,2,4-trichlorobenzene (the typical concentration of saturated solution is around 0.05 mg ml −1 ). Edge chlorination can tune the optical property of GNRs as well. As shown in Fig. 5 , there is obvious colour change between the solution of chlorinated GNRs and pristine GNRs. Both the ultraviolet–visible–near-infrared spectra of chlorinated GNRs and pristine GNRs show the similar absorption features, two absorption peaks (502 and 555 nm for pristine GNRs, and 540 and 591 nm for chlorinated GNRs). The absorption of chlorinated GNRs is red-shifted by 37 nm and exhibits a defined optical band gap (1.7 eV), that is, it is decreased by 0.2 eV compared with pristine GNRs. Taken together, our chlorination protocol enables atomically precise edge functionalization of nanographenes and its application in GNRs, providing well-defined chemical functionalized graphene materials, as an important step towards controlled property modulation. The unambiguous crystallographic characterization of chlorinated nanographenes reveals the structural similarity between nanographenes and infinite graphene, and provides an atomic model for edge-functionalized graphene materials. We demonstrate that precise edge chlorination serves as an efficient approach to modulate the properties of nanographenes, for example, solubility, band gap, energetic position of the frontier molecular orbital and charge transport. This strategy in combination with defined graphene synthesis can lead to designable and uniform graphene materials required by most practical technologies. The chlorine atoms at the edges also provide the opportunity for further chemical derivatization of graphene. Synthesis of 1 A 50-ml flask was charged with 0.1 mmol (52 mg) of C 42 H 18 ( 8 ), 0.2 mmol (26 mg) of AlCl 3 , 30 mmol (5 g ) ICl and 35 ml of CCl 4 , and then the reactants were stirred and refluxed at 80 °C for 48 h. After reaction, the products were poured into 30 ml ethanol to quench the reaction and precipitate the products. Next, the suspension was filtered and the precipitate was washed by ethanol, hydrochloric acid (1.0 mol l −1 ), ion-free water and acetone, sequentially. After dried in vacuum, about 107 mg (0.097 mmol) yellow powder was obtained. The yield of 1 is about 97%. Synthesis of 2 A 50-ml flask was charged with 0.05 mmol (30 mg) of C 48 H 18 ( 9 ), 0.1 mmol (13 mg) of AlCl 3 , 15 mmol (2.5 g ) ICl and 35 ml of CCl 4 , and then the reactants were stirred and refluxed at 80 °C for 48 h. The products were poured into 30 ml ethanol to quench the reaction and precipitate the products. Next, the suspension was filtered. The precipitate was collected and washed by ethanol, hydrochloric acid (1.0 mol l −1 ), ion-free water and acetone, sequentially. After dried in vacuum, about 52 mg (0.043 mmol) orange powder was obtained. The yield of 2 is about 86%. Synthesis of 3 A 50-ml flask was charged with 0.1 mmol (75 mg) of C 60 H 22 ( 10 ), 0.25 mmol (34 mg) of AlCl 3 , 30 mmol (5 g ) ICl and 35 ml of CCl 4 . The reactants were stirred and refluxed at 80 °C for 48 h. Next, the reaction was quenched by ethanol. After that, the excess ICl and CCl 4 were removed by rotary evaporator at 45 °C. The residual solid was washed with ethanol. The product was purified by column chromatography using chloroform as eluent. Compound 3 was collected as the first component at solvent front. After evaporating the solvent, the product was dried in vacuum. About 143 mg (0.095 mmol) dark red powder was obtained. The yield of 3 is about 95%. Synthesis of 4 A 50-ml flask was charged with 0.1 mmol (75 mg) of C 60 H 24 ( 11 ), 0.25 mmol (34 mg) of AlCl 3 , 30 mmol (5 g ) ICl and 35 ml of CCl 4 . The reactants were stirred and refluxed at 80 °C for 48 h, then quenched by ethanol. After that, the excess ICl and CCl 4 were removed by rotary evaporator at 45 °C. The residual solid was washed by ethanol. Next, the product was purified by column chromatography using chloroform as eluent. Compound 4 was collected as the first component at solvent front. After evaporating the solvent, the product was dried in vacuum. About 145 mg (0.093 mmol) red powder was obtained. The yield of 4 is about 93%. Synthesis of 5 A 50-ml flask was charged with 0.05 mmol (60 mg) of C 96 H 30 ( 12 ), 0.20 mmol (28 mg) of AlCl 3 , 30 mmol (5 g ) ICl and 35 ml of CCl 4 . The reactants were stirred and refluxed at 80 °C for 48 h, then quenched by ethanol. After that, the excess ICl and CCl 4 were removed by rotary evaporator at 45 °C. The product was washed by ethanol and then purified by column chromatography using chloroform as eluent. Compound 5 was collected as the first component at solvent front. After evaporating the solvent and dried in vacuum, 100 mg (0.047 mmol) dark violet powder was obtained. The yield of 5 is about 95%. Synthesis of 6 A 50-ml flask was charged with 0.015 mmol (25 mg) of C 132 H 34 ( 13 ), 0.20 mmol (28 mg) of AlCl 3 , 30 mmol (5 g ) ICl and 35 ml of CCl 4 . The reactants were stirred and refluxed at 80 °C for 5 days, and then the reaction was quenched by ethanol. After reaction, the excess ICl and CCl 4 were removed by rotary evaporator at 45 °C. The product was washed with ethanol. Next, the product was purified by column chromatography using chloroform/carbon disulphide (1:1) as eluent. Compound 6 was collected as the first component at solvent front. After evaporating the solvent and dried in vacuum, 34 mg black powder was obtained. The yield of 6 is about 83%. Synthesis of 7 A 50-ml flask was charged with 0.01 mmol (27 mg) of C 222 H 42 ( 14 ), 0.20 mmol (26 mg) of AlCl 3 , 30 mmol (5.0 g ) ICl and 35 ml of CCl 4 . The reactants were stirred and refluxed at 80 °C for 72 h, and then the reaction was quenched by ethanol. After that, the excess ICl and CCl 4 were removed by rotary evaporator at 45 °C. Next, 30 ml ethanol was added. After sonication for 5 min, the suspension was filtered and the precipitate was washed by ethanol. Next, the product was purified by column chromatography using chloroform/carbon disulphide (1:2) as eluent. Compound 7 was collected as the first component at solvent front. After evaporating the solvent and dried in vacuum, 38 mg black powder was obtained. The yield of 7 is about 90%. Synthesis of chlorinated GNRs See Supplementary Methods for experimental details of the synthesis of GNRs and related NMR spectra ( Supplementary Figs S23–S28 ). A 100-ml flask was charged with 25 mg of GNRs, AlCl 3 (26 mg, 0.2 mmol), excess of ICl (5 g , 30 mmol) and 70 ml of CCl 4 , and then the reactants were stirred and refluxed at 80 °C for 4 days. After reaction, 15 ml ethanol was added to quench the reaction. The solvent was removed by rotary evaporator at 50 °C. Next, 30 ml ethanol was added. After sonication for 5 min, the suspension was filtered. The precipitate was washed with ethanol, hydrochloric acid (1.0 mol/l), ion-free water and acetone, sequentially. X-ray single-crystal diffraction characterization of 1 – 5 The single crystals of 1–5 were grown from carbon disulphide solution (compounds 1 and 2 ), carbon disulphide/chloroform (1:1) solution (compound 3 ), toluene solution (compound 4 ) and chloroform/cyclohexane solution (compound 5 ) by solvent evaporation, respectively. The crystals of 1 – 5 were measured on a Stoe diffractometer using a graphite-monochromated Cu Kα radiation source ( 1 ), an Oxford Supernova diffractometer using a graphite-monochromated Cu Kα radiation source ( 2 , 4 and 5 ) and a Bruker diffractometer using a graphite-monochromated Mo Kα radiation source ( 3 ), respectively. Using Olex2 (ref. 33 ), all the initial structures of 1 – 4 were solved with the XS structure solution programme using direct method and refined with the XL refinement package using least-squares minimization [34] . The structure of 5 was solved with the olex2.solve structure solution programme [33] using charge flipping and refined with the XH refinement package using least-squares minimization. Theoretical calculations of chlorinated nanographenes The theoretical calculations of 1 – 7 were carried out at the DFT level, with the Heyd-Scuseria-Ernzerhof (HSE) functional [35] . All stationary points have been optimized and characterized with the 6–31G*Gaussian basis set [36] . Accession codes: The X-ray crystallographic coordinates for structures reported in this article have been deposited at the Cambridge Crystallographic Data Centre (CCDC), under deposition number CCDC 927984 to 927988. These data can be obtained free of charge from CCDC via http://www.ccdc.cam.ac.uk/data_request/cif How to cite this article: Tan, Y.-Z. et al. Atomically precise edge chlorination of nanographenes and its application in graphene nanoribbons. Nat. Commun. 4:2646 doi: 10.1038/ncomms3646 (2013).